Ultrafast viscous water flow through nanostrand-channelled graphene oxide membranes Pressure-driven ultrafiltration membranes are important in separation applications. Advanced filtration membranes with high permeance and enhanced rejection must be developed to meet rising worldwide demand. Here we report nanostrand-channelled graphene oxide ultrafiltration membranes with a network of nanochannels with a narrow size distribution (3–5 nm) and superior separation performance. This permeance offers a 10-fold enhancement without sacrificing the rejection rate compared with that of graphene oxide membranes, and is more than 100 times higher than that of commercial ultrafiltration membranes with similar rejection. The flow enhancement is attributed to the porous structure and significantly reduced channel length. An abnormal pressure-dependent separation behaviour is also reported, where the elastic deformation of nanochannels offers tunable permeation and rejection. The water flow through these hydrophilic graphene oxide nanochannels is identified as viscous. This nanostrand-channelling approach is also extendable to other laminate membranes, providing potential for accelerating separation and water-purification processes. Significant effort has been devoted to the development of highly efficient membrane materials for industrial filtration and separation processes [1] , [2] . Because of their unique physical and chemical properties, nanomaterials have been used to construct novel functional nanostructured membranes [3] , [4] , [5] . Recently, we constructed ultrathin nanoporous membranes with cross-linked protein for ultrafast water permeation [6] and ultrathin diamond-like carbon membranes for fast separation of molecules from organic solvents [7] . Ideally, an efficient ultrafast membrane should be as thin as possible to maximize the permeance, be robust enough to withstand the applied pressure and have a narrow distribution of pore size for excellent selectivity. Graphene is an excellent candidate because of its mono-atomic thickness, two-dimensional structure, high mechanical strength, chemical inertness and impermeability to all gases [8] , [9] , [10] . Theoretical studies have demonstrated that a mono-atomically thick porous graphene membrane exhibits superior separation performance for gases [11] , water [12] and ions [13] , [14] . However, the manufacture of porous graphene membranes on a large scale and the application of such membranes in pressure-driven separation remain challenges [15] , [16] , [17] . Graphene oxide (GO), a functionalized graphene derivative, has recently attracted tremendous attention for its potential use in membrane science because of its facile and large-scale production in solution [18] . Laminated GO-based membranes assembled using micrometre-sized GO sheets exhibit distinguished characteristics, including hydrophilism, outstanding mechanical strength and good flexibility, which make GO an ideal candidate for nanoscale filtration and sieving applications [18] . For example, Geim and co-workers observed that submicrometre-thick free-standing GO membranes were completely impermeable for gases, including He, H 2 , N 2 and Ar. Water vapour, however, permeated through limited capillary channels between pristine graphene regions in the GO membranes, where the hydrophobic graphene wall offers ultralow friction and enables fast water transport [19] . The permeance of water vapour under these conditions is ∼ 0.1 l m −2 ·h −1 ·bar −1 under a pressure of 23 mbar [19] . In addition, Raidongia and Huang [20] and Sun et al. [21] have reported that ions can transport selectively through the fully wetted GO film via diffusion. However, the permeation through these GO membranes remains insufficient to allow them to compete with commercial pressure-driven ultrafiltration membranes because these membranes are limited by their less fluidic channels (the randomly distributed nanoscale wrinkles [20] , [22] and/or spaces strutted by functional hydroxyl, carboxyl and epoxy groups) [21] , [23] and the slow diffusion process therein. Qiu et al. first reported pressure-driven separation performance of the thermally corrugated GO membranes with an elevated permeance of 45 l m −2 ·h −1 ·bar −1 , which was attributed to the presence of microscopic wrinkles in the GO [22] . Nanochannels in the thermally corrugated GO membranes were mainly attributed to microscopic corrugated GO wrinkles. This result implies that the nanochannels in the reconstructed laminated GO membranes, if well defined, are very promising for bona fide nanoscale separation. However, the formation of nanochannels in the aforementioned GO membranes actually cannot be well controlled. Consequently, a percolated nanochannel network with a well-defined channel size within GO membranes is desired to pursue high permeance and selectivity [22] . Here we report the development of ultrafiltration nanostrand-channelled GO (NSC-GO) membranes with numerous nanochannels with diameters of 3–5 nm, superior separation performance of small molecules and ultrafast water permeation (695±20 l m −2 ·h −1 ·bar −1 ). This permeation rate is 10 times higher than that of GO membranes without compromising the rejections and is more than 100 times higher than that of commercial ultrafiltration membranes with similar rejections. Notably, the separation performance exhibits an abnormal dependence on the applied pressure, which is distinctly different from porous polymer filtration membranes and suggests mechanotunable functions [24] , [25] , [26] . On the basis of both experimental and molecular dynamics (MD) simulation results, we determine that this abnormal phenomenon arises from the reversible deformation of the nanochannels in NSC-GO membranes. When the pressure is tuned, these nanochannels experience a series of changes in their shape and cross-sectional area, which, in turn, affect the rejection rates of small molecules and water permeance. Furthermore, the nature of water transporting through the NSC-GO membrane is proven to be classic viscous flow with substantially reduced boundary slip in comparison with that in the plug-like flow confined in the hydrophobic graphene channels, such as single-walled carbon nanotubes [27] and graphene membranes [19] . Synthesis of NSC-GO membranes In this study, GO sheets ( Supplementary Fig. S1a ) were prepared via a modified Hummers’ method (see details in the Methods section), and GO membranes ( Supplementary Fig. S1b ) were prepared using vacuum filtration [18] . The thickness of the membranes was adjusted by tuning the volume of GO suspension to be filtrated. The thicker GO membranes exhibit higher rejection rates of Evans blue (EB, a dye) and lower permeance, as shown in Supplementary Fig. S2 . In addition, considering the uniformity and stability of the membrane, we determine the optimum volume of GO suspension to be 3 ml, which forms membranes with a thickness of ∼ 1,850 nm. As illustrated in Fig. 1 , we prepared NSC-GO membranes were prepared by (1) accumulating a mixed dispersion of the positively charged copper hydroxide nanostrands (CHNs) and negatively charged GO sheets on a porous support; (2) performing a short-time treatment with hydrazine for 15 min; and (3) removing the CHNs using EDTA (see details in the Methods section). The volume of GO suspension filtered can easily control the thickness of the laminar NSC-GO membranes. The positively charged CHNs with a diameter of ∼ 2.5 nm and length up to tens of micrometres ( Fig. 2a ), as prepared using our previous method [28] , assemble tightly with negatively charged GO sheets via electrostatic interaction ( Fig. 2b ) [29] , [30] , [31] . After being filtrated, the CHNs were then incorporated into GO layers. The nanofibrous structures are clearly observed on the surface of the GO/CHNs composite membranes ( Fig. 2c ). Atomic force microscopic (AFM) images ( Supplementary Fig. S3a–c ) further confirm that the CHNs not only attach onto the surfaces of GO sheets but are also intercalated into the stacked GO layers. The height of the nanochannel duplicated by nanostrands is estimated to be ∼ 3.77 nm on the basis of the height profile in Supplementary Fig. S3d,e . The incorporation of CHNs greatly improves the water permeation compared with GO membranes. The preparation of the GO membranes from 3 ml of 0.2 mg ml −1 GO suspension requires 65 min, whereas only ∼ 1 min is required for the formation of a GO/CHNs composite membrane ( Fig. 2d ) via filtration of a mixture of 3 ml of 0.2 mg ml −1 GO and 12 ml of CHN solution. Thus, the CHNs intercalated into GO layers create a network of nanochannels for fast water delivery. 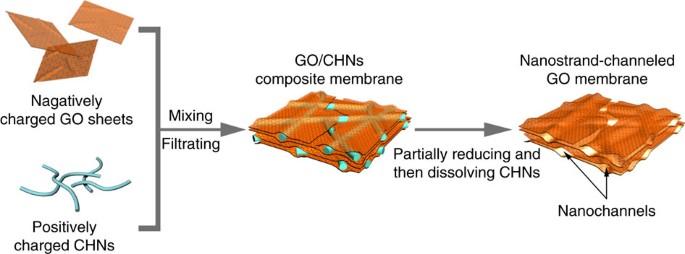Figure 1: Illustration of the fabrication process of NSC-GO membrane. A multi-step process consisting of formation of a dispersion of positively charged copper hydroxide nanostrands (CHNs) and negatively charged GO sheets on a porous support, followed by hydrazine reduction, and finally CHN removal. Figure 1: Illustration of the fabrication process of NSC-GO membrane. A multi-step process consisting of formation of a dispersion of positively charged copper hydroxide nanostrands (CHNs) and negatively charged GO sheets on a porous support, followed by hydrazine reduction, and finally CHN removal. 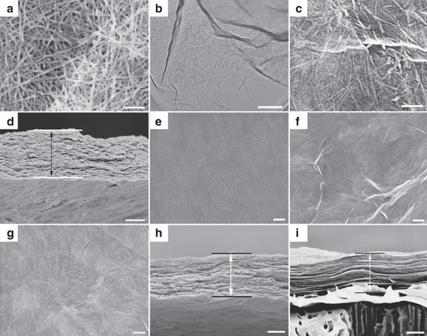Figure 2: Scanning electronic microscopic (SEM) characterizations of GO-based membranes. (a) SEM image of CHNs (scale bar, 200 nm). (b) Transmission electron microscopic image of GO/CHNs composites (scale bar, 500 nm). (c) SEM image of surface of GO/CHNs membrane (scale bar, 100 nm). (d) Side view of GO/CHNs membrane (thickness, 2.17 μm; scale bar, 1 μm). (e) SEM image of GO/CHNs membrane by direct EDTA treatment (scale bar, 200 nm). (f) SEM image of GO/CHNs membrane treated by N2H4for 15 min (scale bar, 100 nm). (g) SEM image of NSC-GO membrane (scale bar, 200 nm). (h) Cross-sectional view of NSC-GO membrane (thickness, 2.03 μm; scale bar, 1 μm). (i) Cross-sectional view of GO membranes (thickness, 1.85 μm; scale bar, 1 μm). Full size image Figure 2: Scanning electronic microscopic (SEM) characterizations of GO-based membranes. ( a ) SEM image of CHNs (scale bar, 200 nm). ( b ) Transmission electron microscopic image of GO/CHNs composites (scale bar, 500 nm). ( c ) SEM image of surface of GO/CHNs membrane (scale bar, 100 nm). ( d ) Side view of GO/CHNs membrane (thickness, 2.17 μm; scale bar, 1 μm). ( e ) SEM image of GO/CHNs membrane by direct EDTA treatment (scale bar, 200 nm). ( f ) SEM image of GO/CHNs membrane treated by N 2 H 4 for 15 min (scale bar, 100 nm). ( g ) SEM image of NSC-GO membrane (scale bar, 200 nm). ( h ) Cross-sectional view of NSC-GO membrane (thickness, 2.03 μm; scale bar, 1 μm). ( i ) Cross-sectional view of GO membranes (thickness, 1.85 μm; scale bar, 1 μm). Full size image To attain a maximum number of nanochannels, membranes with various volume ratios of GO to CHNs ( V GO / V CHNs ) were fabricated and the water permeance through GO/CHNs membranes was measured ( Supplementary Fig. S4 ). The water permeance for the GO/CHN membranes gradually increases with the volume of CHN suspension in the range of 2–12 ml, which indicates that the number of nanochannels increases with increasing CHNs content. However, the permeance almost remains constant as V GO / V CHNs increases to greater than 3:12 because the negative charges on the surface of the GO sheets are balanced with the positively charged nanostrands. Thus, the addition of more CHN cannot create additional nanochannels, and no significant change is observed in the water permeance ( Supplementary Fig. S4 ). Herein, we fixed V GO / V CHNs at 3:12 unless otherwise indicated. Although the GO/CHN membranes exhibit high water permeance, the rejection rate of EB molecules is only 57% ( V GO / V CHNs =3:12), which is much lower than that of GO membrane (85%). The major reason for this low rejection rate is that the inter-sheet spacing is enlarged by the presence of overlapped nanostrands, which is confirmed by X-ray diffraction patterns (i) and (iii) in Supplementary Fig. S5 . The interlayer distance in GO/CHN and GO membranes is 9.86 and 8.49 Å, respectively. To achieve higher rejection rates, the GO/CHNs membranes were immersed in EDTA aqueous solution to dissolve the CHNs within the GO layers. Figure 2e reveals that nanochannels still remain after the CHNs are removed. The energy-dispersive X-ray spectroscopic results ( Supplementary Fig. S6 ) clearly show no detected signal for Cu, thereby indicating the complete removal of the CHNs. However, the membranes here still lack stability and durability during the aqueous separation process. This problem can be solved by partially reducing the GO/CHNs membrane in hydrazine at room temperature and subsequently dissolving the CHNs with EDTA. Figure 2f clearly reveals that the nanofibrous structures still remain after the hydrazine treatment. After the nanostrands have been removed, the linear nanochannels generated by the nanostrands in/on the GO films are distinctly observed, as shown in Fig. 2g . The final NSC-GO membranes have a thickness of 2,030±40 nm ( Fig. 2h ), which is smaller than that of the GO/CHN membrane ( Fig. 2d ) but larger than that of the GO membranes ( Fig. 2i ). This process not only enhances the stability but also mostly reserves the nanochannels because the permeance reaches 695±20 l m −2 ·h −1 ·bar −1 , which is ∼ 1.5 times greater than the value of 451±15 l m −2 ·h −1 ·bar −1 of the membrane after the CHNs were dissolved directly with EDTA. The final NSC-GO membranes are very stable in aqueous separation applications. Nevertheless, this NSC-GO membrane remains hydrophilic and its contact angle with water is 30°. The zeta potential of GO after the hydrazine treatment for 15 min is −40 mV, which is very close to the value of −47 mV for the pristine GO. This result suggests that most of the negatively charged carboxyl groups are retained. As these hydrophilic carboxyl groups are almost on the edges of the GO sheets [18] , specifically, on the entrance of the nanochannels, the condition is favourable for water to access into the nanochannels; indeed, water has been inserted into sub-2 nm carbon nanotubes with hydrophilic open ends at atmospheric pressure [5] . In our case, the pore size of the nanochannels is ∼ 3–5 nm, as determined by the rejection performance (in the next section). Therefore, the NSC-GO membranes could be fully wetted by water and available for aqueous separation. We compared the separation performance of NSC-GO membranes with that of GO membranes. Supplementary Table S1 indicates that the water permeance of the NSC-GO membranes (695±20 l m −2 ·h −1 ·bar −1 ) is 10 times greater than that of GO membranes (71±5 l m −2 ·h −1 ·bar −1 ), whereas the rejection rate for EB is 83±1%, which is almost the same as that of GO membrane (85±2%). These results indicate that these well-defined nanochannels remarkably enhanced the permeance of the NSC-GO membrane without sacrificing their rejection properties. Separation performance of the NSC-GO membranes The separation performance of NSC-GO membranes is typically evaluated by filtrating different types of molecules or ions, including gold nanoparticles (diameter 5 nm), cytochrome c (Cyt. c , 2.5 × 2.5 × 3.7 nm 3 ), EB (1.2 × 3.1 nm 2 ), rhodamine B (RB, 1.8 × 1.4 nm 2 ), 5,10,15,20-tetrakis-( N -methyl-4-pyridyl)-21,23-H-porphyrin tetratosylate (TMPyP, 1.7 × 1.7 nm 2 ), [Fe(CN) 6 ] 3− (diameter 0.9 nm) and neutral molecules γ-cyclodextrin (γ-CD, width <1.2 nm) and γ-CD/adamantane (γ-CD/Ad, 1.2 × 1.2 nm 2 ) at pH ∼ 6.5 (ref. 6 ). The structures of typical dyes or molecules used for the filtration experiments are shown in Supplementary Fig. S7 . Notably, their concentrations are all 1.5 mM or less in the absence of other additional ions. Therefore, the effect of ionic strength can be eliminated [18] . Detailed separation data for the NSC-GO membranes are listed in Table 1 . The NSC-GO membranes demonstrated rejection rates of 20% for γ-CD, 36% for [Fe(CN) 6 ] 3− , 41% for γ-CD/Ad, 83% for EB, 87% for RB, 98% for Cyt. c , 99% for TMPyP and 100% for gold nanoparticles. The ultraviolet–visible absorption results of the feed, the permeate and the retentate are summarized in Supplementary Fig. S8 . Normally, the rejection rate of molecules through nanoporous membranes is dominated by both the molecular-sieving mechanism and electrostatic interactions [1] . However, the zeta potential results indicate that the NSC-GO membrane is negatively charged because of the deprotonation of carboxyl groups on the edges of GO sheets [18] , [32] . Therefore, the rejection of all the negatively charged molecules is dominated by the molecular-sieving mechanism. For example, the rejection rates for negatively charged gold nanoparticles, Cyt. c , EB molecules and [Fe(CN) 6 ] 3− ions are 100, 98, 83 and 36%, respectively, with almost the same permeance ( ∼ 575 l m −2 ·h −1 ·bar −1 ). These size-dependent rejection rates indicate that the effective diameter of the nanochannels is close to the size of EB: 1.2 × 3.7 nm 2 (ref. 6 ). However, given the hydration water layer (0.5 nm) [6] of the GO sheets, the EB and the Cyt. c molecules, the effective pore size of the nanochannels within the NSC-GO membrane is estimated to be 3–5 nm. To understand the effect of the charge characteristics of NSC-GO on molecular sieving, the neutral molecules γ-CD, γ-CD/Ad composite and positively charged molecules RB and TMPyP were examined. Table 1 indicates that the rejection rate is 20% for the flexible γ-CD and increases to 40% for γ-CD filled with Ad. Their permeances are similar to those observed for negatively charged molecules. These observations further confirm the molecular-sieving mechanism. In addition, the negatively charged NSC-GO membranes exhibit 87% rejection and almost 100% rejection for positively charged RB and TMPyP molecules, respectively. However, their permeances are half of those of the neutral and negatively charged molecules previously discussed. This difference cannot be explained by the molecular-sieving effect alone. To eliminate the charge effect, the positively charged molecules feed solution was poured into a separation funnel with the NSC-GO membrane before the filtration until there was no obvious change in the concentration of the feed. We observed that, owing to electrostatic attraction, the negatively charged GO membranes could effectively trap the positively charged RB and TMPyP. As almost all of the negatively charged carboxyl groups are located at the edges of the GO sheets or defects [32] , the entrance of the nanochannels could be partially blocked by the positively charged molecules; thus, the pores are effectively narrowed. This mechanism explains why the rejection rate increases while the permeance decreases for these positively charged molecules. Table 1 Performance evaluation. Full size table To highlight the superior separation performance of the NSC-GO membranes, we compared these membranes with several commercial ultrafiltration membranes under the same experimental conditions. Polysulphone-based ultrafiltration membranes provided by Advantech (Q0100, molecular weight cutoff: 10,000 Da) exhibited a rejection rate of less than 15% for EB and cannot retain small molecules. However, cellulose-based ultrafiltration membranes provided by Millipore (PLCC, nominal molecular weight limit: 5,000 Da) exhibited a rejection rate of 53% for EB with a permeance of 10 l m −2 ·h −1 ·bar −1 , which is 57 times smaller than that of the NSC-GO membranes. Another ultrafiltration membranes from the same company (PLACE, NEWLY 3000) exhibited an 84% rejection rate of EB and a permeance of 4 l m −2 ·h −1 ·bar −1 (ref. 6 ), which is ∼ 144 times lower than that of the NSC-GO membranes. Given that the EB rejection rate of the NSC-GO membranes was ∼ 83%, the permeance was a 100 times higher than that of commercial ultrafiltration membranes with similar rejection rates. Pressure response of the NSC-GO membranes The dependence of the separation performance of NSC-GO membranes on the applied pressure is illustrated in Fig. 3a (blue triangles). The rejection rate for EB molecules is clearly approximately the same ( ∼ 83%) in zone I but continuously decreases to 50% in the zone II. When the pressure increases further, the rejection rate recovers and reaches as high as 95.4% in zone III. This phenomenon is very different from that in polymer-based membranes under the same conditions. In polymer membranes, the rejection rate usually increases with pressure because of the compression and/or densification of their porous structures [24] , [25] , [26] . To explain this unique phenomenon in NSC-GO membranes, we performed measurements of the pressure-dependent water flux through these NSC-GO membranes (the black squares in Fig. 3a ) as an indirect method of exploring the changes in the nanochannels. The results distinctly demonstrate that the flux increases linearly with applied pressure from 0.1 to 0.4 MPa at a rate of 101.1 l m −2 ·h −1 ·bar −1 but increases nonlinearly when the pressure exceeds 0.4 MPa (zone II and III). Both the pressure dependence of the flux and the rejection suggest that, in zone I, no significant change occurs in the nanochannels because of the minimal variation in the rejection and linear flux pressure dependence. The rejection rate then decreases as the pressure increases further from 0.4 to 0.9 MPa (zone II), which suggests an enlarged nanochannel pore size. However, the slope of the flux pressure curve, specifically the permeance decreases, which implies a reduction in the number of nanochannels. These results appear to be paradoxical according to Poiseuille’s law for viscous flow in that the nanochannel size increases while the permeance of the membranes decreases [1] . To understand the underlying mechanism of this unconventional behaviour, we performed MD simulations by modelling a half cylindrical nanochannel in a NSC-GO membrane ( Fig. 3b ) with an effective pore size of ∼ 5 nm and a cross-sectional area of 31 nm 2 . This value is very similar to the cross-sectional area of the nanochannel (34 nm 2 ) we calculated by integrating the marked peak area in Supplementary Fig. S3 . The oxygen-containing groups (including hydroxyl, epoxy and carboxyl groups) were generated by simulating annealing from a randomly assigned structure with oxygen-containing groups on both sides of a graphene sheet (see the details in Methods section). The response of the nanochannel to pressure exertion is illustrated in Fig. 3c–e and in Supplementary Movie 1 , which demonstrates that when a water-filled GO nanochannel is loaded with pressure, its shape changes from round into a flattened rectangle as the pressure is increased to as high as 0.75 MPa. The flattened rectangle is continuously compressed into round ripples as the pressure further increases to as high as 1.5 MPa. These simulation results qualitatively explain the abnormal rejection rate of EB (the blue solid triangles in Fig. 3a ). When the channel is flattened, the cross-sectional area increases from 31 to 41 nm 2 ( Fig. 3b ); thus, the permeation of EB molecules is enhanced significantly. During further compression, consecutive shrinkage of the nanochannels will reduce the cross-sectional area and increase the rejection rate again. The separation performance (flux and rejection rate) of the NSC-GO membranes under repeated pressure loading and unloading was also investigated. Surprisingly, the flux is significantly recovered with a slight increase in the rejection rate in the third pressure-loading round (the red curve in Fig. 3a ). This result indicates that the compressed small nanochannels will almost recover to the original state after the pressure is released, which is reasonable because the strain energy stored in the water-containing curved GO sheets is sufficiently high to overcome the van der Waals forces at the contact region of the newly formed smaller nanochannels [8] , [9] , [10] . In our MD simulations, the compressed nanochannel can quickly recover to its original shape (<0.2 ns). Similar mechanisms have been demonstrated in carbon nanotubes [33] , [34] , [35] , [36] , where the graphene sheet has a bending stiffness (0.91 eV) similar to that of the GO value calculated here (0.85 eV) [37] , [38] . The intercalated guest molecules in the nanochannels, such as water, provide additional elasticity for this reversibility. Our simulation results further indicate that the pore size of the nanochannels could be tuned by controlling the applied pressure, which is consistent with our experimental data. This ability offers a unique and straightforward way for tuning the separation properties of NSC-GO membranes dynamically using applied pressure. 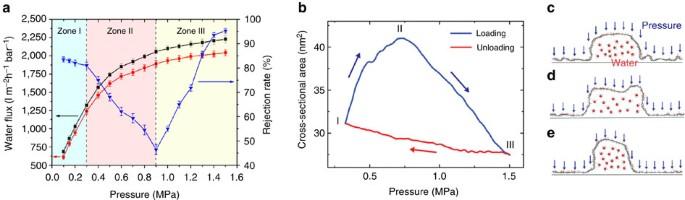Figure 3: Response of NSC-GO membranes to the applied pressure. (a) Pressure-dependent flux and rejection of EB molecules of NSC-GO membrane under different pressure. The black solid squares and red solid circles curve represent the flux variation during the first and third pressure-loading processes, respectively. The blue solid triangle curve denotes the rejection rate of EB during the first pressure-loading process. All the error bars are average errors from five measurement data. (b) Simulated changes in the cross-sectional area of nanochannel by varying the applied pressure. (c–e) The response of a half cylindrical GO nanochannel modelled in MD simulation. Figure 3: Response of NSC-GO membranes to the applied pressure. ( a ) Pressure-dependent flux and rejection of EB molecules of NSC-GO membrane under different pressure. The black solid squares and red solid circles curve represent the flux variation during the first and third pressure-loading processes, respectively. The blue solid triangle curve denotes the rejection rate of EB during the first pressure-loading process. All the error bars are average errors from five measurement data. ( b ) Simulated changes in the cross-sectional area of nanochannel by varying the applied pressure. ( c – e ) The response of a half cylindrical GO nanochannel modelled in MD simulation. Full size image Water vapour has been hypothesized to transfer through the capillaries between pristine graphene regions in GO membranes where the hydrophobic walls offer ultralow friction, which leads to remarkable boundary slip [19] . However, the nature of water flow in the nanochannels within NSC-GO membranes remains an open question. According to our experimental measurements and MD simulation results, we identified the viscous characteristics of water flow through these fully wetted GO nanochannels with hydrophilic surfaces and a uniform size distribution (3–5 nm). As shown in Fig. 3a , the flux of the NSC-GO membranes increases linearly with the applied pressure in zone I, which is typical viscous flow according to the Poiseuille law [1] . In zones II and III, the nonlinear relationship between the water flux and applied pressure arises from the dynamical elastic deformation of the nanochannels, as previously discussed. We further investigated the permeation of the water/ethanol mixture with different viscosities under a pressure of 1 bar. As demonstrated in Fig. 4a , the flux of the water/ethanol mixture with different ratios is inversely proportional to the viscosity. This result indicates that water transports through these nanochannels as viscous flow and obeys Poiseuille’s law [1] . 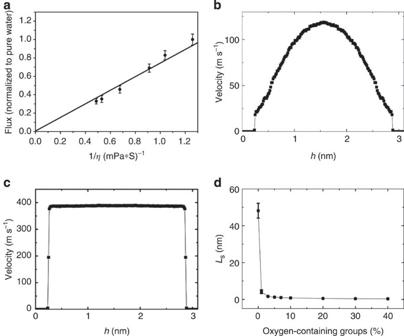Figure 4: Viscous flow through nanochannels within NSC-GO membranes. (a) Flux of various water/ethanol mixtures with different viscosities through the NSC-GO membrane, with the applied pressure at 1 bar. (b,c) Velocity profiles of water flow across a GO channel with oxygen-containing group content of 20% and a pristine graphene channel, respectively. (d) The slip length (Ls) depends on the content of oxygen-containing groups in GO channels. The size of the channels inb–dis 3 nm. Figure 4: Viscous flow through nanochannels within NSC-GO membranes. ( a ) Flux of various water/ethanol mixtures with different viscosities through the NSC-GO membrane, with the applied pressure at 1 bar. ( b , c ) Velocity profiles of water flow across a GO channel with oxygen-containing group content of 20% and a pristine graphene channel, respectively. ( d ) The slip length ( L s ) depends on the content of oxygen-containing groups in GO channels. The size of the channels in b – d is 3 nm. Full size image For membranes with cylindrical pores of a few nanometres in size, viscous flow can be readily described by the Hagen–Poiseuille equation [1] : where J is the flux; ɛ is the surface porosity; r is the pore radius; Δ p is the applied effective pressure; η is the viscosity; d is the membrane thickness and τ is the tortuosity. For the flow between laminated GO membranes, Poiseuille’s law is expressed as (equation (2) in Geim et al. [19] ): where h is the size of the channel in the GO sheets, L is the average lateral length of the GO sheets (1.0 μm in our case), η is the viscosity of water (889 μPa s), and Δ x is the thickness of the GO membrane (2,030 nm). For the laminated GO membranes, h is typically 0.7 nm and the permeance is calculated as ∼ 10 −6 l m −2 ·h −1 ·bar −1 (ref. 19 ). However, for the NSC-GO membrane, h should be determined from the effective pore size (3–5 nm) of the nanochannels in our NSC-GO membranes. Equation (2) thus yields a permeance of 0.94 × 10 −3 l m −2 ·h −1 ·bar −1 , which is five to six orders of magnitude smaller than our experimental measurements (691 l m −2 ·h −1 ·bar −1 for the NSC-GO membranes and 71 l m −2 ·h −1 ·bar −1 for the GO membranes). One possible explanation for this obvious contrast is the presence of many more porous structures in our NSC-GO membranes that undoubtedly generate a much shorter channel length. In equation (2), the ideal porosity of the GO membrane is evaluated by h / L (ref. 19 ), which is only 0.5%. However, in the NSC-GO membrane, the porosity is at least 10 times higher than this value because the thickness of NSC-GO expands to 111% compared with that of GO membranes prepared from the same amount of GO suspension ( Fig. 2h,i ). A second explanation is that due to the high porosity and the defects on the GO sheets [39] , [40] , [41] , the effective channel length in our system is much shorter than the theoretical value ( ∼ 2 mm) calculated from L Δ x / h . Another possibility can be attributed to the enhanced water flow due to the ultralow friction and boundary slip in the nanoconfined hydrophobic channels formed between pristine graphene regions in the GO membranes [19] . In our previous study, we identified plug-like water flow with a distinguished boundary slip flow feature and low friction for water flow between two graphene sheets [38] . In this study, we performed additional MD simulations by substituting the graphene into GO (see details in the Methods section). However, our simulation results reveal that water flow through the nanochannels (3 nm) between GO sheets exhibits a distinct viscous feature. The flow profile of water has a typical parabolic shape ( Fig. 4b ), which contrasts sharply with the plug-like flow with a plateau velocity profile in pristine graphene ( Fig. 4c ), although slight boundary slip still occurs. However, this slip length ( L s ) is significantly reduced by the incorporation of oxygen-containing groups ( Fig. 4d ) of a 3-nm GO channel (see details in Methods section). Typically, the content of oxygen-containing groups in GO prepared by Hummer’s method is ∼ 20% (ref. 41 ). As the zeta potential and the ratio of the I D / I G band are almost the same in the pristine GO and in the GO reduced by N 2 H 4 for 15 min, the density of the oxygen containing groups should be constant. In a 3-nm GO channel with 20% oxygen-containing groups, the slip length ( L s ) in the NSC-GO channels is only 0.35199±0.12735, nm (see details in Methods section), more than two orders of magnitude smaller than the 48±4 nm in a 3-nm graphene channel. On the basis of equation (3) [42] , where ξ is the flow enhancement, Q S is the slip flow rate, Q N is the non-slip flow rate, L S is the slip length and δ is the channel size, the water flow enhancement is ∼ 1.7, which is much smaller than the 82±6 in a 3-nm graphene channel. Therefore, the contribution of the boundary slip to the water flow is negligible in our NSC-GO membranes. In addition, the boundary slip is minimal in a 5-nm GO channel with 20% oxygen-containing groups (as illustrated in Supplementary Fig. S9 ). These findings support our hypothesis related to the mechanism of fluid flow across the NSC-GO membranes because the pore size of the channels within the NSC-GO membrane is 3–5 nm. Water permeating through the NSC-GO membranes can be defined as classic viscous flow with negligible boundary slip, in contrast to the plug-like flow in confined hydrophobic graphene channels, such as single-walled carbon nanotubes [27] and free-standing GO membranes [19] . The high permeance can instead be attributed to both the significant enhancement of the porosity and the much shorter channel length of several micrometres in the NSC-GO membrane. However, technically, direct measurement of the porosity and channel length in fully wetted lamellar NSC-GO membranes remains a huge challenge. In summary, NSC-GO ultrafiltration membranes prepared using a novel nanostrand-channelled strategy exhibit superior pressure-driven separation performance for small molecules. The permeance of NSC-GO membranes is 10 times greater than that of GO membranes without sacrificing rejection rate and is several hundred times higher than that of commercial ultrafiltration membranes with similar rejection rate. Remarkably, the elastic deformation of the nanochannels under pressure leads to an abnormal pressure-dependent separation behaviour, offering a reversibly controllable flux and rejection rate. The water permeating through these GO nanochannels is identified as classic viscous flow with evidence from both experimental and MD simulation results, and the enhancement in water permeance is attributed to the porous structure and reduced channel length. Moreover, the nanostrand-channelling concept introduced in this work could be extended to other porous laminate membranes, enabling the introduction of well-defined and controllable nanochannels for environmental and energy-related applications such as water purification and electrochemical energy storage. Synthesis of GO dispersion The GO sheets were prepared using the modified Hummer’s method as described elsewhere [18] . Graphite powder (0.18 g) was gradually added to a mixture (80 °C) of concentrated sulphuric acid (2 ml), potassium persulphate (0.625 g) and phosphorus pentoxide (0.625 g). The mixture was subsequently maintained at 80 °C in an oil bath under stirring for 4.5 h. Afterwards, the mixture was diluted with an excess of deionized water. The reaction product was collected by vacuum filtration using a 0.2-μm polycarbonate (PC) filter and was subsequently washed with an excess of deionized water to remove the residual acid until the pH value of the filtrate approached to neutrality. The fluffy graphite was dried under ambient condition for 12 h. The dried product was then added to concentrated sulphuric acid (30 ml) at 0 °C with stirring. When the product was fully dispersed, KMnO 4 (3.75 g) was slowly and carefully added. The entire reaction mixture was placed in a water bath at 35 °C for 2 h. Subsequently, the mixture was diluted with 60 ml of deionized water and then reaction was allowed to continue for another 2 h. Then, 175 ml of deionized water was added, followed by a slow addition of 5 ml of 30% H 2 O 2 ; the colour of the dispersed solution immediately changed to brilliant yellow. The solution was centrifuged and washed with 10% HCl solution two or three times. Again it was centrifuged and washed with deionized water at least eight times to fully remove the metal ions and residual acid. The final GO was dried at 60 °C for 2 days. A stable, brownish transparent GO suspension (0.2 mg ml −1 ) was obtained by sonicating 0.2 g of the as-prepared GO in deionized water (1 l) for 2 h. Synthesis of CHNs solution The CHNs were prepared by mixing an equivalent volume of 4 mM Cu(NO 3 ) 2 and 1.4 mM ethanol amine under vigorous stirring for 1 min and then maintaining this mixture at ambient temperature for 1 day [28] . Synthesis of NSC-GO membrane Three millilitres of GO aqueous solution (0.2 mg ml −1 ) with a pH of 6.2 was mixed with 12 ml of CHN solution and stirred for at least 10 min. The mixture was filtered on a PC (Whatman) membrane with a pore size of 0.2 μm, a porosity of 10% and an effective filtration area of 2.83 cm 2 . Subsequently, the GO/CHNs membranes were treated with a diluted hydrazine (15 mM) solution for 15 min, followed by treatment with an EDTA solution to remove the CHNs. Finally, the NSC-GO membranes were obtained. The thickness of the NSC-GO membranes was tunable via the volume of GO and CHN solutions to be filtered. A series of membranes were prepared with V GO / V CHNs of 3:2 to 3:16. Effects of N 2 H 4 treatment The water permeance of the GO/CHNs membrane increases significantly with N 2 H 4 (15 mM) treatment time ( Supplementary Fig. S10 ); however, the EB rejection rate of the corresponding NSC-GO membranes decreases ( Supplementary Fig. S11 ). These variations are attributed to the change in membrane structure. N 2 H 4 is well known to be a strong reducing agent that can easily destroy the layered structure of GO sheets and form structure defects and ripples, as induced by strain when the membrane is exposed to N 2 H 4 for a long time [43] . To evaluate the defects within NSC-GO membranes, Raman spectroscopy—a technique widely used to characterize the structural and other properties of graphene such as disorder and defect structures–was used. The G band is related to the in-plane vibration of sp 2 -bonded carbon atoms, whereas the D band is associated with the vibrations of carbon atoms with sp 3 electronic configurations in disordered graphene [44] . The I D / I G ratio of the NSC-GO membranes as observed in Supplementary Fig. S12 slightly increases with short-time hydrazine treatment, which indicates that the structural defects indeed form in the process of N 2 H 4 treatment and the GO sheets are seldom reduced. Undoubtedly, these structural defects within N 2 H 4 -treated GO/CHNs membranes will apparently affect their water flux. Under these conditions, water and other molecules can easily pass through the membranes through these defects or larger ripples, which will compromise the rejection rate of the final NSC-GO membranes. This effect is not desirable in the design of ultrafast filtration membranes. Therefore, a 15-min hydrazine treatment is ideal for the fabrication of high-separation-performance NSC-GO membranes. Materials characterization X-ray diffraction patterns were obtained using an X’Pert PRO (PANalytical, the Netherlands) diffractometer equipped with a Cu Kα radiation source. The morphologies and structures were characterized using transmission electron microscopy (Tecnai G2 F20 S-TEIN) and field-emission scanning electronic microscopy (Hitachi SU-70) on an instrument equipped with an energy-dispersive X-ray spectrometer. Tapping mode AFM images were obtained using a MultiMode scanning probe microscopy (VEECO). For the AFM observations, the samples were prepared by depositing one droplet of the corresponding samples onto a single crystalline Si substrate that was subsequently dried at room temperature. Evaluation of separation performance A 5-nm gold nanoparticles solution purchased from British Biocell International was diluted 10-fold. Then, 20 ml of the diluted gold solution was filtrated through the as-prepared NSC-GO membranes with effective areas of 2.83 cm 2 on a PC membrane with a 200-nm pore size and 10% porosity using a dead-end filtration cell at room temperature. The gold nanoparticle solutions were neutral. After a certain amount of time, the concentration of the gold nanoparticles in the retentate and permeate were monitored using ultraviolet–visible spectroscopy (SHIMADZU 3600). The separation performances was evaluated on the basis of the amounts of nanoparticles in the retentate, permeate and feed solution. A similar evaluation method was performed for the separation of Cyt. c , EB, RB, TMPyP, [Fe(CN) 6 ] 3− , and neutral molecules γ-CD and γ-CD/Ad. The high-pressure separation experiment was performed using a dead-end separation system (Millipore P158, maximum pressure 1.9 MPa) and high-pressure argon gas. MD simulations MD simulations were performed to evaluate the response of the nanochannels in NSC-GO membranes to the applied pressure and to study the behaviour of water transporting through the NSC-GO membranes. MD simulations were performed using the large-scale atomic/molecular massively parallel simulator package [45] . The reactive force field (ReaxFF) [46] was used to obtain atomic structures and to characterize the properties of GO. All of the simulations were performed using the velocity Verlet integrator with a time step of 0.2 fs. Themostating was implemented by coupling the system under investigation to a Nosé–Hoover thermal bath (at 300 K if not specified otherwise). We modelled the nanochannels by constructing a GO ripple on a graphene substrate. GO sheets were created by randomly distributing epoxy and hydroxyl groups on graphene sheets with the specific chemical composition n C : n H : n O =1:0.12:0.22, where n is the number of atoms. Annealing from 1,000 to 300 K was further simulated to optimize the atomic structures of the GO model. During this process, the surface functional groups relaxed and some of the groups decomposed to free water and other oxygen-containing fragments, which were removed before the subsequent simulations. The nanochannel was modelled by a wrinkled GO sheet deposited on a flat sheet, that is, a half cylinder; the area of the half cylinder was calculated from the space it confined. Within the nanochannels, water molecules were intercalated using the density of water under ambient conditions. The amount of water was adjusted to obtain a nanochannel size comparable to that in our experiments. To explore the structural distortion, we applied pressure in the simulations by external forces on the atoms in GO. During the pressure loading on the GO membrane in our experiments, fluid flow was driven across the percolated network consisting of both the interlayer space between the GO sheets and the nanochannels created by dissolving the nanostrands. Thus, the pressure asserted on the GO sheet could be simulated via the application of force in the direction perpendicular to the GO plane, as used in our MD simulations. We explored the interfacial slippage of water between the GO walls. To quantify the slippage, we calculated the solid–liquid friction coefficient ( λ ) from the frictional force autocorrelation function according to the Green–Kubo formula: where F x ( t ) is the time-dependent total force acting on a surface with area S , which could be then related to the slip length ( L s ) through L s = η / λ (refs 47 , 48 ). A shear viscosity η =0.729 mPa·s (for the extended simple point charge water model at 300 K, which can be enhanced in a nanoconfined environment) was used for the confined water in the evaluation. The optimized all-atom force field optimized potentials for liquid simulations all-atomic was used here for GO to save computation time, and the van der Waals interaction between water and GO was described using the Lennard–Jones formula with parameters ɛ =4.063 eV and σ =0.319 nm [49] , [50] . We verified this set of parameters by successfully reproducing the experimentally measured contact angle, that is, θ C =29.1° with 20% oxygen-rich functional groups. The results for the slip length are plotted in Fig. 3d , which indicate that the slip length of water flow between pristine graphene sheets is 48 nm and is reduced drastically by two orders of magnitude to 0.35 nm for GO with 20% oxygen-containing groups. With the hydroxyl functionalization, not only is the boundary slip suppressed, as measured by the reduction of L s , but the nature of the flow is also modified. To characterize this phenomenon, we simulated pressure-driven water flow by applying direct forces onto water molecules. This non-equilibrium MD approach has been widely used to explore fluid flow [8] . As demonstrated in Fig. 3b , a parabolic velocity profile is obtained for the water flow inside a GO nanochannel, which is dramatically different from the plug-like flow with a plateau velocity profile within the pristine graphene nanochannel [38] , [42] . The implementation of a pressure gradient across the channel should be assessed, as noted in the literature such as in the paper by Docherty et al. [51] To validate our results, we performed a new set of simulations with minimal computation. In the new model, forces were applied to a selected region (2 nm in a 12.28-nm long channel, which can be considered as the inlet or outlet as the periodic boundary conditions were applied) instead of to all of the water molecules. The results (see Supplementary Figs S13 and S14 ) indicate that the implementation of driven pressure quantitatively causes a difference in the velocity profile (with the maximum velocity of 100 m s −1 for the new model instead of 119 m s −1 for the one presented in the main text for GO channels and much less (<2.5%) for graphene channels), the qualitative picture does not change and our conclusion about the nature of viscous flow remains valid. How to cite this article: Huang, H. et al. Ultrafast viscous water flow through nanostrand-channelled graphene oxide membranes. Nat. Commun. 4:2979 doi: 10.1038/ncomms3979 (2013).